Roquin binding to target mRNAs involves a winged helix-turn-helix motif Roquin proteins mediate mRNA deadenylation by recognizing a conserved class of stem-loop RNA degradation motifs via their Roquin domain. Here we present the crystal structure of a Roquin domain, revealing a mostly helical protein fold bearing a winged helix-turn-helix motif. By combining structural, biochemical and mutation analyses, we gain insight into the mode of RNA binding. We show that the winged helix-turn-helix motif is involved in the binding of constitutive decay elements-containing stem-loop mRNAs. Moreover, we provide biochemical evidence that Roquin proteins are additionally able to bind to duplex RNA and have the potential to be functional in different oligomeric states. Binding of proteins to distinct cis -regulatory elements within the untranslated region (UTR) of messenger RNAs (mRNAs) regulates the lifespan of these mRNAs and controls the gene expression at the post-transcriptional level. Roquin proteins, for example, were recently reported to specifically bind to a newly discovered conserved class of RNA stem-loop motifs, known as constitutive decay elements (CDE), which are present in the 3′ UTR of various mRNAs, thereby initiating their degradation. On a transcriptome-wide scale, >50 vertebrate CDE-containing mRNAs were identified as Roquin targets, many of which encode proteins important for development as well as inflammation and immunity [1] . Roquin binding to the CDE in the 3′ UTR of tumour necrosis factor-α (TNF-α) mRNA, for example, limits the synthesis of the proinflammatory cytokine TNF-α (ref. 1 ). The expression of ICOS (inducible T-cell costimulator), a gene encoding an essential receptor for follicular T-cells, is also restricted by Roquin, which promotes the degradation of ICOS mRNA, thereby playing an important role in autoimmunity [2] , [3] . Mammalian genomes encode two roquin paralogs with seemingly redundant functions [4] , [5] . Human ROQUIN1, also known as RC3H1 (ring finger and CCCH-type zinc finger domains 1), is a 1,133 amino-acid protein, containing a RING (really interesting new gene)-type zinc finger, a roquin domain (ROQ), a CCCH-type zinc finger (zf), and a poorly defined carboxy (C)-terminal, proline-rich domain. Murine Roquin binding to CDE-like RNA stem-loop motifs was shown to be mediated by the ROQ domain, while the C-terminal effector domain recruits the Ccr4–Caf1–Not complex, resulting in Caf1a-dependent deadenylation and consecutive degradation of CDE-containing mRNAs [1] . Although Roquin proteins were shown to act broadly as mediators of mRNA deadenylation by recognizing a conserved class of stem-loop RNA degradation motifs via the ROQ domain [1] , the structural basis for stem-loop mRNA recognition is still unknown. To shed light on this, we determined the crystal structure of the ROQ domain of the human ROQUIN1 protein revealing a winged helix-turn-helix (wHTH) motif. Additional biochemical and mutational analyses show that ROQUIN1 is able to bind both stem-loop and duplex RNA and that these interactions are mediated by the wHTH motif. Moreover, we provide evidences that ROQUIN1 has the potential to be functional in various oligomeric states and also provide a dimer model of the ROQ domain. Crystal structure of the ROQ domain To obtain the crystal structure of the human ROQUIN1/RC3H1 protein, several constructs were used for crystallization. Although the produced proteins comprised up to three functional domains (RING, ROQ, zf domains), we always obtained the same degradation product, most likely representing the ROQ domain with all stably folded elements. We determined the crystal structure of this portion of ROQUIN1 at 1.91-Å resolution by single-wavelength anomalous diffraction phasing. 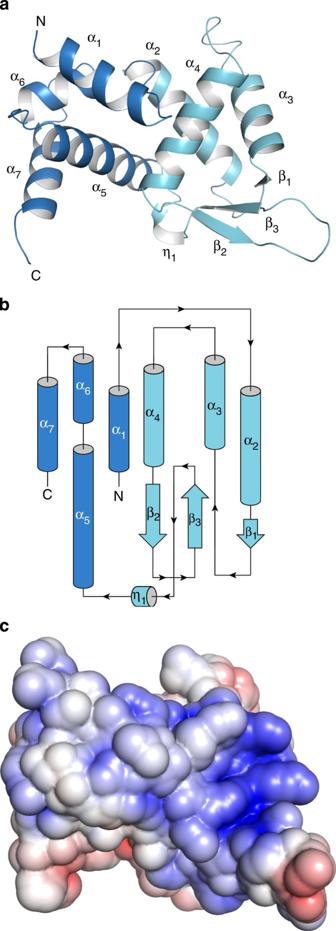Figure 1: Crystal structure of the ROQ domain of ROQUIN1. (a) Cartoon model of the overall fold with the wHTH motif highlighted in light blue. (b) Topological model of the ROQ domain fold. Colouring in panelsaandbis identical. (c) The electrostatic surface of the ROQ domain (orientation as ina), calculated with the APBS plugin in Pymol (±5 kT/e; red, negative; blue, positive). The final model was refined to an R work of 20.0% and an R free of 24.1% ( Table 1 , Supplementary Fig. 1a,b ) and includes amino-acid residues 177–328. The overall structure of the ROQ domain shows a compact (α+β) fold featuring seven α-helices, one 3 10 -helix and a short three-stranded antiparallel β-sheet ( Fig. 1a ). The structure reveals a wHTH motif spanning from helix α2 to the 3 10 -helix η1, with helix α1 and helices α5–α7 from the ROQ domain packing against the wHTH motif ( Fig. 1a,b , Supplementary Fig. 1a ). The overall fold is stabilized by a salt bridge between the wHTH motif (R251 in helix α4) and a C-terminal residue of helix α5 (E293), and by hydrogen bonding interactions between the amino (N)-terminal helix α1 and helices α2 and α4 of the wHTH motif. Table 1 Data collection, phasing and refinement statistics. Full size table Figure 1: Crystal structure of the ROQ domain of ROQUIN1. ( a ) Cartoon model of the overall fold with the wHTH motif highlighted in light blue. ( b ) Topological model of the ROQ domain fold. Colouring in panels a and b is identical. ( c ) The electrostatic surface of the ROQ domain (orientation as in a ), calculated with the APBS plugin in Pymol (±5 kT/e; red, negative; blue, positive). Full size image The canonical wHTH motif has originally been described to bind double-stranded DNA and consists of three α-helices (H1–H3), three β-strands (S1–3) and two characteristic loops (‘wings’) W1 and W2, arranged in the order H1-S1-H2-H3-S2-W1-S3-W2 (ref. 6 ). Notably, in the crystal structure of the ROQ domain, the wHTH motif adopts a similar conformation with the exception that the W2-loop of the canonical wHTH motif is folded into the single-turn 3 10 -helix η1 ( Fig. 1a,b ). Moreover, the putative RNA-binding pocket is located within the wHTH motif as illustrated by electrostatic potential mapping ( Fig. 1c ). Currently, the wHTH motif is described as a conserved structural element whose interaction profiles and functional properties in different proteins are extremely versatile, ranging from nucleic acid binding to protein–protein interactions [6] . Search for structural homologues using the DALI server [7] and PDBeFold [8] returned no matches for the entire structure but to other wHTH-containing protein domains, whereby sharing a sequence identity of only 10–15%, explaining the missed wHTH motif prediction. The DNA replication factor Cdt1 (PDB code 3a4c (ref. 9 )), a key licensing factor that recruits the MCM2–7 complex onto the origin of chromosomes, is the closest structural homologue with a root-mean-square deviation (r.m.s.d.) of 3.2 Å over 99 α-carbons ( Supplementary Fig. 2a ). Other structural similarity matches identified by the DALI [7] search were wHTH domains found in E3 ubiquitin ligase complexes. The complex of the C-terminal domain of cullin-1 and the RING domain of the E3 ubiquitin ligase Rbx1 (ref. 10 ), for example, superimposes with an r.m.s.d. of 3.8 Å over 79 residues onto the wHTH motif of the ROQ domain ( Supplementary Fig. 2b ). In the cullin–RING ligase complex, the wHTH subdomain of cullin-1 mediates contacts with the Rbx1 RING domain and similar interactions might be observed between the wHTH motif of the ROQ domain and the N-terminal RING domain of ROQUIN1. Notably, no matches to other proteins with classical wHTH motifs and reported RNA-binding properties were found among the top hits in the structural similarity search [7] . However, to date only few such proteins have been described, displaying diverse RNA recognition modes [11] , [12] , [13] , [14] , [15] , [16] . Among these, the selenocysteine tRNA-specific elongation factor SelB is the single example of a wHTH-containing protein recognizing stem-loop mRNA. Its C-terminal domain encompasses four wHTH domains. The two terminal tandem wHTH motifs synergize to establish specific interactions with the selenocysteine incorporation site hairpin, and the last motif specifically recognizes the mRNA-specific hairpin tip structure of the mRNA [12] , [16] . The C-terminal SelB wHTH domain superimposes with an r.m.s.d. of 3.1 Å over 73 residues onto the wHTH motif within the crystal structure of the ROQ domain, displaying a similar electropositive pocket as described for the ROQ domain crystal structure ( Supplementary Fig. 2c ). ROQUIN1 binding to CDE-containing stem-loop mRNAs Structural analysis indicated a role of the wHTH motif of the ROQ domain in RNA binding. To support this finding, we analysed the RNA-binding properties of different wHTH variants. Within the wHTH motif, single basic residues that may confer binding of the RNA backbone are highly conserved throughout the Roquin homologues. However, clusters of basic solvent-accessible residues can be found at the N-terminal base of helix α3 (R219 and K220) and in the β2–β3 loop (K259 and R260) ( Supplementary Fig. 3 ). To verify a potential involvement of these wHTH residues in mRNA binding, we performed electrophoretic mobility shift assays (EMSA) using wild-type and variant proteins comprising the RING, ROQ and zf domains of ROQUIN1 (RC3H1 2–452 ), and the isolated CDE-containing stem-loop structure of ICOS mRNA. Wild-type RC3H1 2–452 binds with a K d value of 139±42 nM to ICOS stem-loop mRNA ( Fig. 2a ), which is comparable with the binding constant reported for another CDE-containing stem-loop mRNA, namely TNF-α (92±14 nM) [1] . On the other hand, RC3H1 2–452 variants with single basic patch mutations (RK219AA or KR259AA, respectively) showed significantly reduced ICOS binding while simultaneous mutation of the two basic patches nearly abolished binding ( Fig. 2a ), clearly demonstrating an involvement of the wHTH motif in stem-loop mRNA binding. Notably, the observed effects are not due to altered secondary structures induced by the mutation as demonstrated by circular dichroism (CD) spectroscopy measurements ( Supplementary Fig. 4 ). 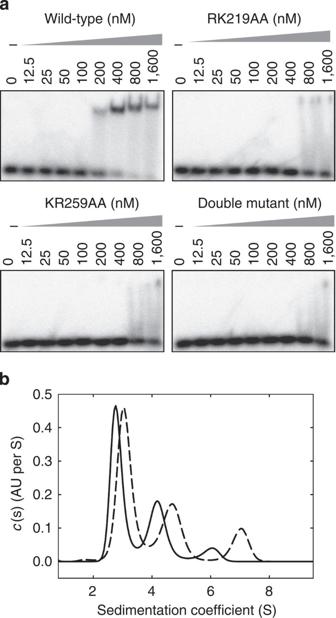Figure 2: ROQUIN1 stem-loop ICOS-mRNA binding studies. (a) EMSA experiments performed with the isolated CDE stem-loop structure of ICOS mRNA and wild type or variant RC3H12–452. The double mutant corresponds to RK219AA/KR259AA of RC3H12–452. The results are representative of at least two independent experiments. (b) Analytical ultracentrifugation analyses of uncomplexed (—) and stem-loop ICOS RNA-complexed (---) RC3H12–452protein. Figure 2: ROQUIN1 stem-loop ICOS-mRNA binding studies. ( a ) EMSA experiments performed with the isolated CDE stem-loop structure of ICOS mRNA and wild type or variant RC3H1 2–452 . The double mutant corresponds to RK219AA/KR259AA of RC3H1 2–452 . The results are representative of at least two independent experiments. ( b ) Analytical ultracentrifugation analyses of uncomplexed (—) and stem-loop ICOS RNA-complexed (---) RC3H1 2–452 protein. Full size image Stem-loop RNA binding to dimeric ROQUIN1 ROQUIN1 purified as monomeric protein as judged by its gel filtration profile. To verify the oligomerization state in solution, we additionally performed sedimentation velocity ultracentrifugation experiments with the RC3H1 2–452 protein, revealing the presence of 60% monomers, 33% dimers and 7% higher oligomers ( Fig. 2b ). This points towards the ability of ROQUIN1 to bind to RNA in various oligomerization states. To shed light on this, we next repeated the experiment in the presence of stem-loop ICOS RNA. All protein peaks are shifted to higher sedimentation coefficients on complex formation with RNA with no significant changes in the relative abundance of the various species, supporting the above hypothesis ( Fig. 2b ). Analysis of the analytical ultracentrifugation experiments indicated that, in addition to monomeric protein, also ROQUIN1 dimers are able to bind to stem-loop RNA. Inspection of the ROQ domain crystal structure and adjacent symmetry-related segments by using ePISA [17] revealed a potential dimer arrangement ( Fig. 3a ) that could allow for independent binding of two stem-loop RNA molecules to the two electropositive wHTH sites within the dimer ( Fig. 3b ), assuming that the stem-loop RNA-binding sites are identical in monomeric and dimeric ROQUIN1. Moreover, we consider this crystallographic dimer rather weak per se as indicated by the small buried surface area of 738 Å 2 with a limited number of hydrogen bonding and salt-bridge interactions at the dimer interface ( Supplementary Table 1 ), and the fact that the dimeric fraction of uncomplexed ROQUIN1, whose existence has been indicated by our analytical ultracentrifugation experiments ( Fig. 2b ), is not stable under the separation shear forces on a gel filtration ( Supplementary Fig. 5a ). 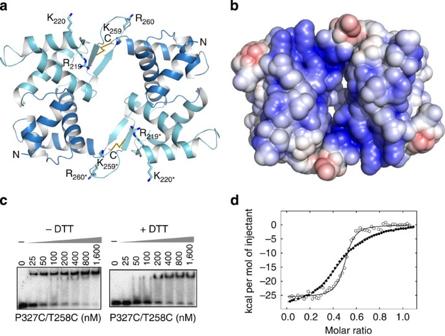Figure 3: Model of the dimeric ROQ domain, capable to bind to various RNA forms. (a) Cartoon model of the dimeric ROQ domain with the wHTH motif highlighted in light blue. Amino acids involved in RNA binding are labeled and shown in stick representation. Dimer-stabilizing disulfide bonds, generated by the P327C/T258C mutation, are shown in yellow. (b) The electrostatic surface of the dimeric ROQ domain (orientation as in panela), calculated with the APBS plugin in Pymol (±5 kT/e; red, negative; blue, positive). (c) EMSA performed with the P327C/T258C variant of the RC3H12–452protein and the isolated CDE stem-loop structure of ICOS mRNA. The results are representative of at least two independent experiments. (d) ITC isotherms characterizing the binding of wild type and P327C/T258C RC3H12–452protein to duplex ICOS RNA. The data were fitted to a one-site binding model, revealingKdvalues of 68.9±8.6 nM and 724.6±20.9 nM and stoichiometry values ofn=0.499±0.003 andn=0.469±0.002 for wild-type and cysteine-bridged dimer of RC3H12–452, respectively, with errors referring to the s.e. of the fit. Figure 3: Model of the dimeric ROQ domain, capable to bind to various RNA forms. ( a ) Cartoon model of the dimeric ROQ domain with the wHTH motif highlighted in light blue. Amino acids involved in RNA binding are labeled and shown in stick representation. Dimer-stabilizing disulfide bonds, generated by the P327C/T258C mutation, are shown in yellow. ( b ) The electrostatic surface of the dimeric ROQ domain (orientation as in panel a ), calculated with the APBS plugin in Pymol (±5 kT/e; red, negative; blue, positive). ( c ) EMSA performed with the P327C/T258C variant of the RC3H1 2–452 protein and the isolated CDE stem-loop structure of ICOS mRNA. The results are representative of at least two independent experiments. ( d ) ITC isotherms characterizing the binding of wild type and P327C/T258C RC3H1 2–452 protein to duplex ICOS RNA. The data were fitted to a one-site binding model, revealing K d values of 68.9±8.6 nM and 724.6±20.9 nM and stoichiometry values of n =0.499±0.003 and n =0.469±0.002 for wild-type and cysteine-bridged dimer of RC3H1 2–452 , respectively, with errors referring to the s.e. of the fit. Full size image To verify that this proposed dimer is capable of stem-loop RNA binding, we designed a dimer-stabilizing mutant and introduced two disulfide bridges at the dimer interface by generating the P327C/T258C variant, which links the C terminus of the ROQ domain to the C-terminal end of β2 within the wHTH motif. The double-cysteine variant purifies as a mixture of monomers and dimers, with the dimeric fraction being convertible to monomers on DTT treatment ( Supplementary Fig. 5b ) and with a secondary-structure content similar to wild-type protein ( Supplementary Fig. 4 ). Strikingly, the disulfide-stabilized dimer possesses a significantly increased stem-loop RNA affinity compared with wild-type protein as revealed by EMSA ( Fig. 3c ). Addition of DTT brings the RNA-binding ability back to wild-type level ( Fig. 3c ), supporting our proposed dimer model. ROQUIN1 binding to duplex RNA To further analyse the stoichiometry of RNA binding to ROQUIN1, we performed isothermal titration calorimetry (ITC) where we calculated an unexpected overall binding stoichiometry of around 0.5, implying that two molecules of RC3H1 2–452 protein bind to one molecule of RNA ( Fig. 3d ). However, we realized that the concentrations applied during this ITC experiment involved RNA annealing at a rather high concentration yielding bulged duplex RNA instead of the stem-loop form ( Supplementary Figs 5c and 6 ), a phenomenon that has also been described by Tan et al . [18] Interestingly, we determined a K d value of 68.9±8.6 nM for the binding of RC3H1 2–452 to ICOS duplex RNA ( Fig. 3d ), which is in the same range as observed for stem-loop RNA. Taken together, ROQUIN1 is not only able to bind to stem-loop but also to double-stranded RNA. Results from analytical gel filtration experiments confirmed the 2:1 binding model indicated by the above ITC experiment. In the absence of duplex RNA, the calculated molecular mass corresponds to monomeric RC3H1 2–452 protein, and the dimeric protein was found in the presence of duplex ICOS RNA ( Supplementary Fig. 5a ). Notably, we observe a complete shift of the monomeric fraction on duplex RNA addition despite adding only 0.6-fold molar amount of duplex RNA to prepare the complex. The same holds true also for the crystallized RC3H1 178–328 degradation fragment of ROQUIN1, indicating that the RING and zf domains of ROQUIN1 are dispensable for both RNA binding and dimerization ( Supplementary Fig. 5d ). The latter finding hints towards the possibility that the proposed ROQ domain dimer arrangement ( Fig. 3a ) may also support duplex RNA binding. In accordance with the 2:1 binding stoichiometry and the electrostatic potential mapping ( Fig. 3b ), the putative duplex RNA-binding site is likely located at the dimer interface. Furthermore, the width of the binding groove at the dimer interface seems sufficient to accommodate double-stranded RNA. To prove our hypothesis, we performed an ITC experiment using the cysteine-bridged P327C/T258C variant of RC3H1 2–452 . Remarkably, a ROQUIN1 dimer stabilized this way binds to ICOS duplex RNA with the same 2:1 stoichiometry as described before (when referring to monomer protein in ITC calculations), substantiating the dimer model ( Fig. 3d ). Compared with wild type, the observed ~10-fold decreased K d value for duplex ICOS binding to the stabilized ROQUIN1 dimer variant may be attributed to the decrease of flexibility in the rigidified cysteine-bridged dimer, which otherwise may be necessary for efficient duplex RNA binding at the dimer interface ( Supplementary Fig. 7a ). Since the two basic patches within the wHTH motif contribute to the electropositive surface at the dimer interface, we next tested whether a variant with simultaneous mutation of these sites (RK219AA and KR259AA) would also interfere with duplex ICOS binding. Indeed, this variant nearly abolished duplex RNA binding ( Supplementary Fig. 8 ), demonstrating that the wHTH motif within the ROQ domain is not only involved in stem-loop RNA binding but also has the potential to recognize double-stranded RNA. Finally, we examined whether the ROQ domain dimerization is mediated predominantly by duplex RNA binding or by monomer–monomer contacts. ITC experiments show that the RC3H1 2–452 variant proteins bearing mutations in the dimer interface bind double-stranded ICOS RNA with similar affinity as wild-type ROQUIN1 ( Supplementary Fig. 8 ). This observation supports a model where ROQUIN1 dimers are formed following duplex RNA binding. The capability of wHTH-containing proteins to bind to duplex RNAs at the interface of the two monomers has also been described for Zα domain-containing proteins that play a role in antiviral responses by recognizing foreign nucleic acids in the cytoplasm [19] . Its wHTH motif contacts five phosphates of a left-handed duplex Z-RNA with residues from its H3 recognition helix and the W1-loop [13] . Moreover, two Zα domains interact with the RNA duplex without forming a physical dimer, suggesting a cooperative mode of RNA-binding [19] . Our work provides insight into the mode of RNA binding by ROQUIN1. Combined structural and biochemical analyses substantiate the involvement of the wHTH motif of the ROQ domain in CDE-containing stem-loop mRNA binding. Furthermore, we illustrate that ROQUIN1 is additionally able to bind to double-stranded RNA and has the potential to be functional in various oligomerization states. Notably, the ROQ domain of ROQUIN1 appears to be sufficient both for RNA binding and dimerization. Finally, we propose a dimer model of the ROQ domain that accounts for stem-loop as well as duplex RNA binding. During revision of this manuscript, two independent publications appeared describing structural aspects of roquin–RNA interactions [18] , [20] . The findings of these authors are in general agreement with the data presented here, particularly with regard to the involvement of the wHTH motif in CDE-containing stem-loop RNA binding [18] , [20] , the ability of the ROQ domain to bind also RNA duplexes [18] and to dimerize, either concentration-dependent [20] or induced by duplex RNA binding [18] . The dimeric arrangement seen in the crystal structure of the ROQ domain bound to duplex RNA [18] differs from our proposed dimer model. This difference may be attributed to the use of a different and longer RNA molecule, namely CDE-containing TNF23, in that study compared with the present work. To examine whether our dimer model is also relevant for TNF ds RNA binding, we performed EMSA experiments with the disulfide-stabilized P327C/T258C dimer variant of RC3H1 2–452 that again displays an increased affinity compared with wild-type protein ( Supplementary Fig. 9a ). Addition of DTT to disrupt disulfide links brings the dsRNA binding affinity back to wild-type level ( Supplementary Fig. 9a ). To rule out unspecific binding of the TNF ds RNA duplex, we finally tested the cysteine-bridged RC3H1 2–452 dimer for binding of the single-stranded RNA species of TNF ds , which almost abolished binding, indicating the requirement of a duplex nature of the RNA for efficient binding by ROQUIN1 ( Supplementary Fig. 9b ). Conclusively, multiple modes of interaction with RNA might be possible, depending on the nature of the RNA (see also Supplementary Fig. 7b ). Whether the described dimeric states of Roquin proteins are physiologically relevant remains to be demonstrated. As indicated by our analytical ultracentrifugation experiments, monomeric ROQUIN1 predominates at lower protein concentrations, but a concentration-dependent dimerization of Roquin has been reported by Schlundt et al . [20] Since Roquin proteins accumulate in P bodies and stress granules [3] , [21] , it is tempting to speculate that elevated Roquin concentration at these sites might favour the formation of functional dimers. In conclusion, Roquin proteins turn out to be very versatile in terms of the secondary structure of their bound RNA targets. It is conceivable that in addition to the reported CDE-containing stem-loop mRNAs also other structure-sequence motifs are recognized within targeted mRNAs, as also indicated by the fact that the majority of the mRNAs enriched in RC3H1 immunoprecipitation experiments were lacking the CDE motif [1] . This opens up exciting prospects for future research, addressing further biological roles of Roquin family members. Cloning, expression and purification DNA encoding the RING, ROQ and zf domains of human ROQUIN1 (RC3H1 2–452 , aa 2–452), the RING and ROQ domains (RC3H1 2–399 , aa 2–399), the ROQ domain (RC3H1 53–399 , aa 53–399) and the crystallized ROQ domain (RC3H1 178–328 , aa 178–328) was subcloned into the pQLinkH vector [22] . The following primers were used for cloning: RC3H1_2fw 5′- CAGGATCCCCTGTACAAGCTCCACAATGG -3′, RC3H1_53fw 5′- GAG GAT CCG ACC AGA CCA CTA TCA ATA CAG ACA -3′, RC3H1_178fw 5′- GAG GAT CCC AAC TCT CTT CCA ATC TTT GGG C -3′, RC3H1_328rv 5′- GAC TGA CTG CGG CCG CTC AGG CTG GAG TCT GCA ACT TG -3′, RC3H1_399rv 5′- GAC TGA CTG CGG CCG CTC AGC TGT GGT TCT GGA TAT AAT CAA CC -3′, and RC3H1_452rv 5′- GAC TGA CTG CGG CCG CTC AGC GCT TAT TCA TTT TAC GAA ATT TTT CC -3′. Mutants were generated using the QuikChange Site-Directed Mutagenesis Kit (Stratagene) according to the manufacturer’s protocol. The genes were expressed as N-terminal His 7 -tagged proteins at 17 °C in E. coli Rosetta 2 (DE3) (Novagen) using a LEX ultra-high-throughput bench-top bioreactor (Harbinger Biotech). Cells were grown at 37 °C in Terrific Broth medium and induced at an OD 600 of 2.0–2.5 with 0.5 mM isopropyl β- D -1-thiogalactopyranoside. For purification, cells were resuspended in PBS lysis buffer (1 × PBS pH 7.4, 0.5 M NaCl, 5% (v/v) glycerol, 0.5 mM dithiothreitol (DTT)), supplemented with 0.25% (w/v) 3-[(3-cholamidopropyl)dimethylammonio]-1-propanesulfonate, 0.1 mM phenylmethyl sulfonyl fluoride, 1 U ml −1 RNase-free DNase I (Qiagen) and one tablet of EDTA-free Complete Protease Inhibitor (Roche). The purification protocol comprises mechanical cell lysis by sonication (SONOPULS HD 2200, Bandelin), Ni/Zn affinity chromatography on a 5 ml HisTrap FF crude column (GE Healthcare) and size-exclusion chromatography on a Superdex 200 prep grade column (XK 26 × 60, GE Healthcare). The His 7 tag was cleaved with tobacco etch virus protease before the gel filtration step, followed by a reapplication of the cleaved protein on the Ni/Zn affinity column. The purification of protein constructs comprising the RING, ROQ and zf domains additionally included a cation-exchange chromatography on a Source 30S column (HR 16 × 10, GE Healthcare). The P327C/T258C variant was expressed in E. coli SHuffle express cells (NEB), and the buffers for initial purification steps included 3 mM GSH (glutathione) and 0.6 mM GSSG (glutathione disulfide). Protein crystallization The ROQ domain was crystallized using the sitting-drop vapour-diffusion method at 20 °C by mixing equal volumes (200 nl) of His 7 tag cleaved RC3H1 2–399 or RC3H1 53–399 protein (8.5 or 10 mg ml −1 in 20 mM HEPES/NaOH pH 7.5, 0.2 M NaCl, 5 mM DTT, ±1 mM (NH 4 ) 2 PtCl 4 ) and reservoir solution (Pt derivative: 16% w/v PEG 6000, 10 mM sodium citrate; native: 20% (w/v) PEG 6000, 0.2 M lithium chloride, 0.1 M Tris/HCl pH 8.0). Before flash-freezing in liquid nitrogen, the crystal was transferred into a cryoprotectant consisting of reservoir solution supplemented with 30% (v/v) glycerol. For derivatization, 0.2 μl 0.5 M (NH 4 ) 2 PtCl 4 ) was added to the crystallization drop before transfer to the cryoprotectant. Data collection, structure determination and refinement Diffraction data were collected on BL14.1 operated by the Helmholtz-Zentrum Berlin (HZB) at the BESSY II electron storage ring (Berlin-Adlershof, Germany) [23] at wavelengths of 1.0727 or 0.9184 Å, respectively. Data were processed with the program XDSAPP [24] . Platinum derivative crystals were used for phasing by single-wavelength anomalous diffraction. Two peak data sets collected from the same crystal were merged with XSCALE [25] to increase multiplicity. The platinum substructure was solved using HKL2MAP [26] , and the phases derived from the identified platinum positions were used for density modification as implemented in the PHENIX AutoSol wizard [27] . Autobuilding of an initial model and refinement were done with PHENIX [28] . The graphics program COOT [29] was used for model building and visualization. The resulting model was transferred to the high-resolution native data by molecular replacement using the program P HASER [27] and refined with REFMAC [30] . Data collection and refinement statistics are reported in Table 1 . The Ramachandran map produced by MolProbity [31] shows that 98.7% of the modelled residues are in favoured regions with no outliers. Structure evaluation Secondary-structure elements were assigned using the program DSSP [32] . Searches for similar structures were performed with PDBeFold [8] and the DALI -Server [7] . Interfaces present in the crystal were analysed using the web service ePISA [17] . Molecular drawings were created with PyMOL Molecular Graphics System (Version 1.3, Schrödinger, LLC). APBS was used for calculating electrostatic surface potentials [33] . Multiple sequence alignment Amino-acid sequences were aligned using the Clustal Omega server [34] , and TEXshade [35] was used for illustration. Uniprot accession numbers are as follows. RC3H1: Homo sapiens , Q5TC82; Mus musculus , Q4VGL6; Rattus norvegicus , D3ZKG8; Gallus gallus , E1BZI9; Xenopus laevis , Q6NUC6. RC3H2: Homo sapiens , Q9HBD1; Mus musculus , P0C090; Rattus norvegicus , D3ZBM2; Gallus gallus , F1NZ02. Roq: Drosophila melanogaster , Q9VV48. Isothermal titration calorimetry ITC measurements were performed at 15 °C in 20 mM Tris/HCl, pH 8.0 and 60 mM KCl using a VP-ITC microcalorimeter (MicroCal Inc.). Before the measurement, protein and synthetic RNA (ICOS_13nt: 5′- AUUUC UGUGA AAU -3′ (Biomers); annealed at about 750 μM) were dialysed against this buffer. Experiments were performed by injecting 55 × 5 μl of 75–100 μM duplex ICOS RNA solution into a sample cell containing 15–20 μM wild-type or variant of RC3H1 2–452 . Injections were performed with a spacing of 240 s and a reference power of 18 μcal s −1 . Integration of the injection peaks and construction of binding isotherms was performed by using the high-precision automated peak shape analysis software NITPIC 1.0.3 (ref. 36 ). Data analysis was performed with the Origin 7.0 software (MicroCal, USA) using a one-site binding model. Analytical gel filtration Absolute molecular masses of the proteins and RNA complexes were determined by analytical gel filtration using a calibrated 10/300 Superdex 200 column. The running buffer contained 20 mM HEPES/NaOH, pH 7.5 and 0.1 M NaCl. For each protein sample, 50–100 μl of a 1–5 mg ml −1 protein solution was applied. RNA complexes were prepared by adding the 0.6-fold amount of duplex ICOS_13nt RNA (annealed at about 750 μM) to the protein. The P327C/T258C mutant of RC3H1 2–452 was analysed with/without 30 min preincubation with 100 mM DTT at room temperature. Circular dichroism spectroscopy Wild-type or variant RC3H1 2–452 proteins were dialysed against 10 mM sodium phosphate buffer pH 7.5 and 20 mM NaF and diluted to 2 μM. Spectra were recorded in three replicates at 20 °C from 260 nm to 185 nm, with a 0.1 nm step size using a Chirascan CD spectrophotometer (Applied Photophysics). Electrophoretic mobility shift assay The EMSA experiments were performed according to Ryder et al . [37] with the following modifications: RNA was prepared by 5′ end-labelling of commercially synthesized RNA oligonucleotides with [γ- 32 P]-ATP using T4 polynucleotide kinase (NEB). Labeled RNA was gel-purified, eluted and adjusted with water to 0.5 pmol μl −1 . 350 fmol of labeled RNA was used per 20 μl reaction. Before binding reactions, a master mix containing labeled RNA, 1 × binding buffer (20 mM Tris-HCl pH 7.5, 50 mM KCl, 5 mM MgCl 2 , 20 μM ZnSO 4 , 10% glycerol), 2 mM DTT and 0.05 mg ml −1 BSA was heated at 90 °C for 1 min and gradually cooled down to room temperature. In parallel, a dilution series of 10 × protein stock was prepared in 1 × protein dilution buffer (1 × binding buffer, 5 μg ml −1 heparin). For each binding reaction, 2 μl of the 10 × protein stock was added to 18 μl of the master mix at room temperature for 2–3 h. After addition of 4 μl 6 × loading buffer (30% glycerol, bromphenol blue, xylene cyanol), RNP complexes were resolved by non-denaturing PAGE (6% polyacrylamide, 0.5 × TBE, 5% glycerol) in ice-cold 0.5 × TBE buffer containing 20 μM ZnSO 4 at 100 V for 40 min. The protein-bound RNA and the free RNA were imaged using a phosphorimager. The P327C/T258C mutant of RC3H1 2–452 was analysed with/without 30 min preincubation with 10 mM DTT at room temperature. The results are representative of two to four independent experiments. For K d calculation, the average of bound fraction from three independent experiments was normalized to the total signal for each lane and plotted against the protein concentration. The data points were fitted by nonlinear regression with errors referring to the s.e. of the fit. Analytical ultracentrifugation Sedimentation velocity experiments were carried out at 35,000 r.p.m. in an XLI analytical ultra-centrifuge (Beckman). For all samples, 400 μl of RC3H1 2–452 protein at a concentration of 0.3 mg ml −1 ±1.1-fold excess of stem-loop ICOS RNA (annealed at 2 μM) and reference buffer (20 mM Hepes pH 7.5, 0.1 M NaCl) were loaded in two-channel center pieces with an optical path length of 12 mm. Samples were measured at 15 °C in an An-50 Ti rotor using the interference optical system. The program SEDNTERP was used to estimate the partial specific volume from amino-acid composition as well as the density ρ and viscosity η of the buffer at 15 °C ( http://bitcwiki.sr.unh.edu/index.php/Main_Page ). Data were then analysed with the program SEDFIT [38] using a continuous c(s) distribution model. Theoretical sedimentation coefficients for monomeric and higher oligomeric protein species were calculated using the following equation with N A Avogadro’s number and M W and f / f 0 the protein’s molecular weight and frictional ratio, respectively. Assuming a frictional ratio of 1.5, sedimentation coefficients of 2.8, 4.4 and 5.8 or 2.9, 4.6, and 6.1 were calculated for monomeric, dimeric or trimeric uncomplexed protein or protein–RNA complexes, respectively. The monomeric uncomplexed protein has a molecular weight of 50.9 kDa for monomers, the monomeric protein–RNA complex is about 55 kDa. How to cite this article : Schuetz, A. et al . Roquin binding to target mRNAs involves a winged helix-turn-helix motif. Nat. Commun. 5:5701 doi: 10.1038/ncomms6701 (2014). Accession codes: Coordinates and structure factors for the ROQ domain of human RC3H1/ROQUIN1 have been deposited in the Protein Data Bank under accession code 4ULW .